Small molecule-mediated stabilization of vesicle-associated helical α-synuclein inhibits pathogenic misfolding and aggregation α-synuclein is an abundant presynaptic protein that is important for regulation of synaptic vesicle trafficking, and whose misfolding plays a key role in Parkinson’s disease. While α-synuclein is disordered in solution, it folds into a helical conformation when bound to synaptic vesicles. Stabilization of helical, folded α-synuclein might therefore interfere with α-synuclein-induced neurotoxicity. Here we show that several small molecules, which delay aggregation of α-synuclein in solution, including the Parkinson’s disease drug selegiline, fail to interfere with misfolding of vesicle-bound α-synuclein. In contrast, the porphyrin phtalocyanine tetrasulfonate directly binds to vesicle-bound α-synuclein, stabilizes its helical conformation and thereby delays pathogenic misfolding and aggregation. Our study suggests that small-molecule-mediated stabilization of helical vesicle-bound α-synuclein opens new possibilities to target Parkinson’s disease and related synucleinopathies. Parkinson’s disease is the second most common neurodegenerative disease. It is characterized by specific movement disturbances and affects ~1% of the population above 60 years [1] . Pathologically, Lewy bodies constitute the hallmark of the disease [2] . Lewy bodies are intraneuronal aggregates formed by misfolded species of the presynaptic protein α-synuclein (αSyn), as well as a multitude of proteins and lipids [3] , [4] , [5] , [6] , [7] . So far, only symptomatic treatment is available for Parkinson’s disease and related synucleinopathies. Although the normal function of αSyn is still a matter of debate, recent evidence suggests that αSyn is important for regulation of synaptic vesicle trafficking and neurotransmitter release via SNARE–complex interaction [1] , [8] , [9] , [10] . Under physiological conditions, αSyn is found in equilibrium between a free monomeric species, which samples a large ensemble of dynamic conformations [11] , [12] , [13] , and a membrane-bound α-helical structure [14] , [15] , [16] , [17] , [18] , [19] . αSyn preferentially interacts with acidic phospholipids [20] where it folds into a single continuous helix extending up to approximately residue 100 (refs 21 , 22 ). In line with the membrane-induced folding of αSyn, two antiparallel, surface-bound helices are formed in the presence of detergent micelles [8] , [23] , [24] . When αSyn is bound to vesicles, the highly aggregation-prone non-amyloid component (NAC) region (residues 61–95), is in an α-helical conformation and acts as a membrane sensor [25] . Since the NAC region is important for initiating αSyn misfolding and forms the core of amyloid fibrils [26] , stabilization of the helical, vesicle-bound conformation of αSyn might interfere with pathogenic aggregation. Increasing evidence indicates that the most toxic species of αSyn are soluble oligomeric aggregation intermediates [10] , [27] , [28] , [29] . The search for small chemical compounds that interfere with the aggregation of unfolded, monomeric αSyn into toxic oligomers and fibrils has therefore been intensively pursued using a wide array of in vitro and cellular systems as well as animal models of Parkinson’s disease [30] , [31] , [32] , [33] , [34] , [35] , [36] , [37] . In contrast, little is known about inhibition of αSyn aggregation in the physiological environment of a vesicle. Indeed, interaction with membranes does not inhibit the potentially pathological process of αSyn aggregation, but can even promote it [20] , [38] . Moreover, perturbation of the membrane integrity by αSyn, potentially resulting in formation of membrane pores, was suggested to cause neuronal death [39] . Here we demonstrate that several small molecules that were previously shown to delay aggregation of soluble, disordered αSyn, are not able to inhibit aggregation of vesicle-bound αSyn. In contrast, the polyphenol phtalocyanine tetrasulfonate (PcTS) directly binds to vesicle-bound αSyn, stabilizes its helical conformation and inhibits misfolding and aggregation. We further show that PcTS prevents inclusion formation and toxicity in a cell model of αSyn aggregation. Thus, our study opens novel possibilities for interfering with αSyn misfolding and neurotoxicity in its physiological environment. PcTS stabilizes the helical structure of lipid-bound αSyn A multitude of organic compounds from different chemical classes were shown to modulate aggregation of αSyn in solution [30] , [31] , [32] , [33] , [40] . This includes the polyphenols curcumin, baicalein and epigallocatechin gallate (EGCG), the drug selegiline, which is used for treatment of early-stage Parkinson’s disease, and the porphyrin PcTS ( Fig. 1a ). In agreement with previous studies, curcumin, baicalein and EGCG inhibited almost completely the formation of αSyn fibrils in solution when used at a 15:1 compound-to-protein ratio ( Supplementary Fig. 1 ). Selegiline and PcTS reduced ThT staining to a smaller degree ( Supplementary Fig. 1 ). PcTS was previously shown to favour prefibrillar αSyn species [34] . 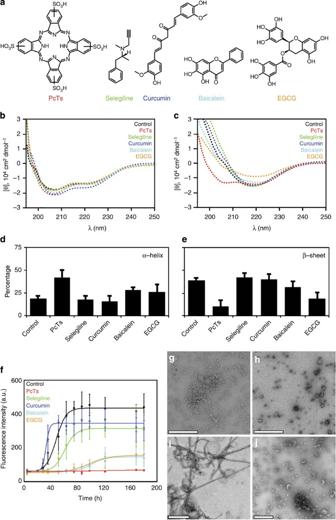Figure 1: A small organic molecule stabilizes vesicle-bound αSyn and inhibits its aggregation. (a) Chemical structure of PcTS, selegiline, curcumin, baicalein and EGCG. (b,c) Circular dichroism spectra of αSyn before (b) and after incubation for 10 days in aggregation-prone conditions (c), both in the absence and presence of a 15:1 excess of PcTS (red), selegiline (green), curcumin (blue), baicalein (light blue) and EGCG (orange). The lipid-to-protein molar ratio was 125:1. In the presence of PcTS, the α-helix content was ~41% and less than 10% of β-structure was formed after 10 days of incubation in aggregation-prone conditions. (d–f) α-helix (d) and β-sheet (e) content together with ThT fluorescence (f) aggregation kinetics of vesicle-bound αSyn. The control did not contain any small molecule. Error bars represent ±s.d. from the mean of at least three different experiments. As the C-terminal domain remains disordered in vesicle-bound αSyn13, the maximum α-helical content is ~70%. InwtαSyn fibrils, the central domain (approximately residues 38–96 with some loops) is converted into β-structure60, corresponding to a β-structure content of ~40%. (g–j) Electron micrographs of fresh (g,h) and aggregated (i,j) αSyn/SUV samples: control (g,i) and PcTS (h,j). The white bar represents 500 nm. Figure 1: A small organic molecule stabilizes vesicle-bound αSyn and inhibits its aggregation. ( a ) Chemical structure of PcTS, selegiline, curcumin, baicalein and EGCG. ( b , c ) Circular dichroism spectra of αSyn before ( b ) and after incubation for 10 days in aggregation-prone conditions ( c ), both in the absence and presence of a 15:1 excess of PcTS (red), selegiline (green), curcumin (blue), baicalein (light blue) and EGCG (orange). The lipid-to-protein molar ratio was 125:1. In the presence of PcTS, the α-helix content was ~41% and less than 10% of β-structure was formed after 10 days of incubation in aggregation-prone conditions. ( d – f ) α-helix ( d ) and β-sheet ( e ) content together with ThT fluorescence ( f ) aggregation kinetics of vesicle-bound αSyn. The control did not contain any small molecule. Error bars represent ±s.d. from the mean of at least three different experiments. As the C-terminal domain remains disordered in vesicle-bound αSyn [13] , the maximum α-helical content is ~70%. In wt αSyn fibrils, the central domain (approximately residues 38–96 with some loops) is converted into β-structure [60] , corresponding to a β-structure content of ~40%. ( g – j ) Electron micrographs of fresh ( g , h ) and aggregated ( i , j ) αSyn/SUV samples: control ( g , i ) and PcTS ( h , j ). The white bar represents 500 nm. Full size image Next, we tested whether curcumin, selegiline, baicalein, PcTS and EGCG interfere with the binding and folding of αSyn on the surface of small unilamellar vesicles (SUVs) [21] . To address this question, we formed SUVs from a 1:1 mixture of 1-palmitoyl-2-oleoyl phosphatidylcholine (POPC) and 1-palmitoyl-2-oleoyl phosphatidic acid (POPA). NMR spectroscopy showed that selegiline, baicalein and EGCG interact with POPA/POPC liposomes ( Supplementary Fig. 2 ). Nevertheless, none of the compounds impaired vesicle binding of αSyn and its folding into an α-helical conformation even at a 15-fold excess of compound with respect to αSyn ( Fig. 1b and Supplementary Fig. 3 ). Are the small molecules able to modulate the aggregation of αSyn in the presence of vesicles? To address this question, αSyn was subjected to aggregation-promoting conditions (37 °C, constant stirring) for 10 days in the absence and presence of the small molecules. When no compound was present, the α-helical content of αSyn decreased from ~70% to below 25% ( Fig. 1b–d ). In parallel, β-structure was formed, the sample stained for the amlyoid-dye thioflavin T (ThT) and electron microscopy revealed fibrillar structures ( Fig. 1c,e,f,i ), consistent with previous results [1] , [34] , [41] . Despite its strong antiaggregation capacity towards soluble αSyn ( Supplementary Fig. 1 ), curcumin did not block the transition from α-helix to β-structure of vesicle-bound αSyn nor the formation of amyloid fibrils ( Fig. 1c–f and Supplementary Fig. 4 ). Selegiline, baicalein and EGCG also did not interfere with the loss of α-helical structure ( Fig. 1c,d ), although samples aggregated in the presence of EGCG and baicalein stained only weakly for ThT, probably as a result of competition with the compounds for binding sites on αSyn fibrils ( Fig. 1f ). The amount of fibrils observed in EM micrographs in the presence of EGCG was small ( Supplementary Fig. 4 ), indicating that EGCG directs αSyn into off-pathway aggregates both in solution [32] and in the presence of vesicles. Curcumin, baicalein, selegiline and EGCG were used at a 15:1 compound-to-protein ratio. The reported apparent binding constants of curcumin and baicalein to αSyn are 10 μM and 500 nM, respectively, while selegiline does at best bind weakly to monomeric αSyn, but interacts with oligomeric species [30] , [31] , [33] , [42] , [43] . In contrast to curcumin, selegiline, baicalein and EGCG, no ThT signal was detected after 10 days of incubation of vesicle-bound αSyn when PcTS was present ( Fig. 1f ). In addition, EM micrographs were free of fibrillar structures and the vesicle morphology appeared unmodified ( Fig. 1h,j ). Quantification of the secondary structure indicated that even after 10 days of incubation in aggregation-prone conditions the α-helix content remained at ~41% and less than 10% of β-structure was formed ( Fig. 1c–e ). Thus, PcTS is able to stabilize the helical, membrane-bound conformation of αSyn and inhibit its aggregation in the presence of vesicles. PcTS also inhibited αSyn aggregation in the presence of large unilamellar vesicles (LUVs; Fig. 2 ). Experiments at different αSyn:compound ratios further showed that a 5:1 but not a 1:1 PcTS:αSyn ratio was sufficient to inhibit amyloid formation ( Supplementary Fig. 5 ). 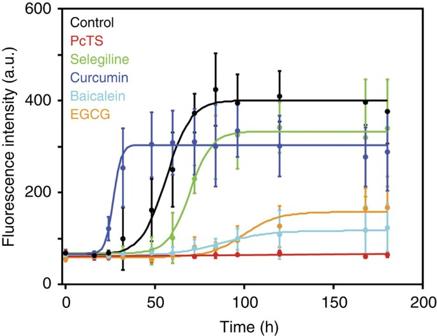Figure 2: Influence of selected small molecules on αSyn fibril formation in the presence of large unilamellar vesicles. Fibril formation kinetics in aggregation-prone conditions (37 °C with stirring). The concentration of αSyn was 100 μM. Fifteenfold excess of compound over protein was used. The final DMSO concentration was 1% of the total volume. Average values of at least three different samples. Error bars represent ±s.d. from the mean of at least three different experiments. Figure 2: Influence of selected small molecules on αSyn fibril formation in the presence of large unilamellar vesicles. Fibril formation kinetics in aggregation-prone conditions (37 °C with stirring). The concentration of αSyn was 100 μM. Fifteenfold excess of compound over protein was used. The final DMSO concentration was 1% of the total volume. Average values of at least three different samples. Error bars represent ±s.d. from the mean of at least three different experiments. Full size image PcTS releases the NAC region from the vesicle surface To obtain insight into the mechanism of the stabilization of the α-helical structure of membrane-bound αSyn by PcTS, we used solution NMR spectroscopy. Although the slow tumbling rate of vesicles induces lipid-bound αSyn to exhibit dynamic properties that hamper its direct observation by solution NMR, exchange with the NMR-visible, lipid-free form allows residue-specific access to the properties of the membrane-bound state [24] . We probed this exchange process using two-dimensional 15 N– 1 H heteronuclear single quantum coherence (HSQC) experiments of 100 μM αSyn in the presence of 12.5 mM SUVs (1:125 protein-to-lipid ratio). In line with previous studies [24] , the NMR signal intensities of the 100 N-terminal residues were strongly decreased compared with free αSyn ( Fig. 3a red spectrum; 3b, red line). The observed signal originates from unbound αSyn, as the bound protein does not contribute [24] . In the C-terminal region, the NMR resonances had a comparable intensity as in the free state, indicating that they interact at best weakly with vesicles. 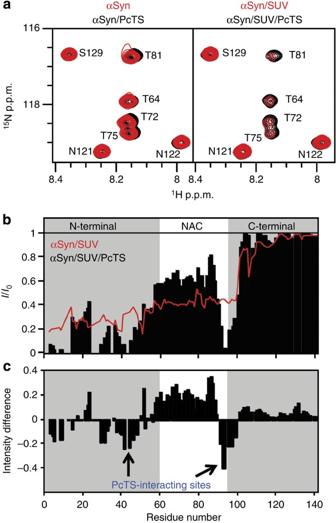Figure 3: PcTS binding partially releases the αSyn NAC region from vesicles. (a) Selected region of 2D15N–1H HSQC spectra of free (left) and vesicle-bound αSyn (right) in the absence (red) and presence of a 15-fold excess of PcTS (black). NMR signals of residues in the NAC region are significantly broadened when in contact with liposomes (right panel). Upon PcTS addition (black spectrum), cross-peaks of these amino acids gain in intensity, indicating a partial release from the vesicle surface. (b) Quantification of NMR signal intensities along the αSyn sequence when bound to SUVs in the absence (red line) and presence of a 15-fold excess of PcTS (black bars). Signal intensities (I) were normalized by the values observed for αSyn in the absence of SUVs (I0). The lipid-to-protein molar ratio was 125:1. White colour marks the aggregation-prone NAC region (residues 61–95). Note that when residues are no longer in contact with liposomes, they become ‘visible’ to solution NMR. (c) Quantification of the signal intensity difference upon addition of PcTS. The intensity decrease around Y39 and F94 is because of the binding of PcTS in free αSyn. Figure 3: PcTS binding partially releases the αSyn NAC region from vesicles. ( a ) Selected region of 2D 15 N– 1 H HSQC spectra of free (left) and vesicle-bound αSyn (right) in the absence (red) and presence of a 15-fold excess of PcTS (black). NMR signals of residues in the NAC region are significantly broadened when in contact with liposomes (right panel). Upon PcTS addition (black spectrum), cross-peaks of these amino acids gain in intensity, indicating a partial release from the vesicle surface. ( b ) Quantification of NMR signal intensities along the αSyn sequence when bound to SUVs in the absence (red line) and presence of a 15-fold excess of PcTS (black bars). Signal intensities ( I ) were normalized by the values observed for αSyn in the absence of SUVs ( I 0 ). The lipid-to-protein molar ratio was 125:1. White colour marks the aggregation-prone NAC region (residues 61–95). Note that when residues are no longer in contact with liposomes, they become ‘visible’ to solution NMR. ( c ) Quantification of the signal intensity difference upon addition of PcTS. The intensity decrease around Y39 and F94 is because of the binding of PcTS in free αSyn. Full size image Upon addition of 1.5 mM PcTS (15:1 compound-to-protein ratio), the cross-peaks of residues in proximity to Y39 and F94 as well as at the N terminus were further attenuated and shifted ( Fig. 3a–c and Supplementary Fig. 6 ). The intensity decrease and chemical shift changes are caused by the binding process and were previously observed upon addition of PcTS to soluble αSyn [34] . It shows that PcTS is in solution and can bind to the residual unbound protein. In contrast, residues within the NAC region (residues 61–95) gained ~20–30% of intensity ( Fig. 3a , black spectrum; Fig. 3b , black bars; Fig. 3c ). In addition, at higher lipid-to-protein ratios, when no NMR signals are observed for the N-terminal 100 residues, addition of PcTS led to the appearance of resonances from the NAC region ( Supplementary Fig. 7 ). Thus, PcTS promotes a faster exchange of the NAC region between the vesicle-bound and free state, making NAC residues ‘visible’ in the NMR spectrum. Using a different buffer system (50 mM phosphate, pH 7.4) and/or different liposome composition (1,2-dioleoyl- sn -glycero-3-phosphoethanolamine (DOPE), 1,2-dioleoyl- sn- glycero-3-phospho- L -serine (DOPS) and 1,2-dioleoyl- sn -glycero-3-phosphocholine (DOPC) in a 5:3:2 ratio) yields the same behaviour in which the NAC region of αSyn is released from its interaction with the membrane ( Fig. 4 ). In addition, the concentrations of PcTS used here are not sufficiently large to interfere with the formation of liposomes ( Supplementary Fig. 8 ). In contrast to PcTS, addition of curcumin, selegiline and baicalein did not change the NMR signal intensity profile of αSyn in the presence of POPC/POPA vesicles ( Fig. 5 ). EGCG further reduced the NMR signal intensity of residues 1–130, consistent with the EGCG-mediated conversion of αSyn molecules, which are not bound to the vesicles, into off-pathway oligomeric species. 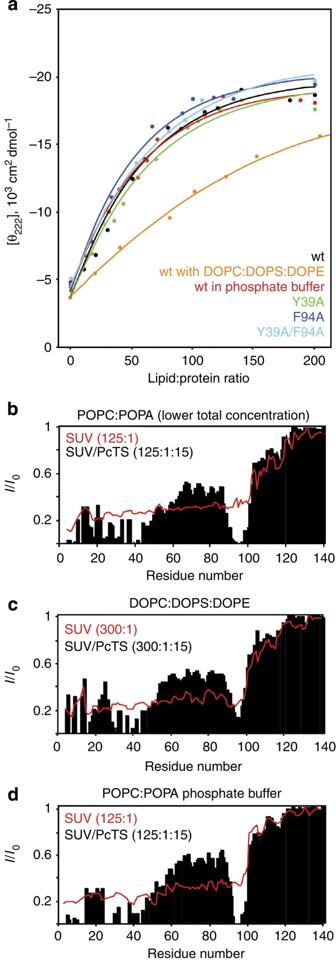Figure 4: Influence of mutations and buffer/lipid composition on αSyn vesicle binding. (a) The mean residue ellipticity at 222nm of αSyn variants for increasing lipid-to-protein ratios. When not indicated otherwise, SUVs were composed of a 1:1 mixture of POPA:POPC and the buffer system was 5 mM HEPES buffer, 10 mM NaCl, pH 7.4. In addition, data for the wild-type protein in 5 mM sodium phosphate buffer, 10 mM NaCl (red) are shown. The Y39A, F94A and Y39A/F94A mutations do not attenuate αSyn's binding to liposomes (a; green, blue and cyan, respectively). (b–d) Quantification of NMR signal intensities along the αSyn sequence when bound to SUVs in the absence (red line) and presence of a 15-fold excess of PcTS (black bars). Signal intensities (I) were normalized by the values observed for αSyn in the absence of SUVs (I0). (b) When compared withFig. 3b, the same molar ratios of αSyn:SUVs:PcTS were used, but at an overall fivefold decreased concentration (2.5 mM SUVs, 20 μM αSyn, 300 μM PcTS). The lipid-to-protein molar ratio was 125:1. (c) NMR signal-broadening profile in the presence of vesicles composed of DOPE, DOPS and DOPC at a molar ratio of 5:3:2. Because of the lower affinity of αSyn to DOPE:DOPS:DOPC vesicles (when compared with POPA:POPC vesicles) a higher lipid-to-protein ratio was used. (d) Effect of PcTS on the liposome-induced NMR signal-broadening profile of αSyn in a 50mM sodium phosphate buffer containing 10 mM NaCl, pH 7.4. SUVs were composed of a 1:1 mixture of POPA:POPC. NMR measurements were performed at 15 °C. Figure 4: Influence of mutations and buffer/lipid composition on αSyn vesicle binding. ( a ) The mean residue ellipticity at 222nm of αSyn variants for increasing lipid-to-protein ratios. When not indicated otherwise, SUVs were composed of a 1:1 mixture of POPA:POPC and the buffer system was 5 mM HEPES buffer, 10 mM NaCl, pH 7.4. In addition, data for the wild-type protein in 5 mM sodium phosphate buffer, 10 mM NaCl (red) are shown. The Y39A, F94A and Y39A/F94A mutations do not attenuate αSyn's binding to liposomes ( a ; green, blue and cyan, respectively). ( b – d ) Quantification of NMR signal intensities along the αSyn sequence when bound to SUVs in the absence (red line) and presence of a 15-fold excess of PcTS (black bars). Signal intensities ( I ) were normalized by the values observed for αSyn in the absence of SUVs ( I 0 ). ( b ) When compared with Fig. 3b , the same molar ratios of αSyn:SUVs:PcTS were used, but at an overall fivefold decreased concentration (2.5 mM SUVs, 20 μM αSyn, 300 μM PcTS). The lipid-to-protein molar ratio was 125:1. ( c ) NMR signal-broadening profile in the presence of vesicles composed of DOPE, DOPS and DOPC at a molar ratio of 5:3:2. Because of the lower affinity of αSyn to DOPE:DOPS:DOPC vesicles (when compared with POPA:POPC vesicles) a higher lipid-to-protein ratio was used. ( d ) Effect of PcTS on the liposome-induced NMR signal-broadening profile of αSyn in a 50mM sodium phosphate buffer containing 10 mM NaCl, pH 7.4. SUVs were composed of a 1:1 mixture of POPA:POPC. NMR measurements were performed at 15 °C. 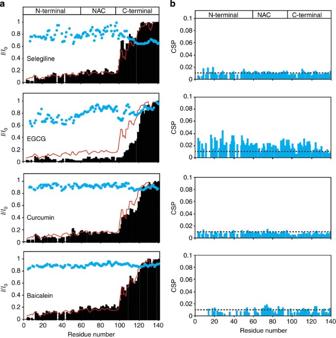Figure 5: Interaction of small molecules with soluble and vesicle-bound αSyn. (a) Quantification of NMR signal intensities along the αSyn sequence when bound to SUVs in the absence (red line) and presence of a 15-fold excess of selegiline, EGCG, curcumin and baicalein (black bars). Signal intensities (I) were normalized by the values observed for αSyn in the absence of SUVs (I0). The lipid-to-protein molar ratio was 125:1. The ratio of NMR signal intensities of free (in the absence of SUVs) αSyn in the presence and absence of the respective compound are shown in light blue. (b) Chemical shift differences for free αSyn in the absence and presence of the compounds. EGCG causes intensity and chemical shift changes because of its binding to monomeric αSyn and conversion of αSyn into off-pathway oligomers. The dashed lines represent the intrinsic error for the chemical shift measurement. Full size image Figure 5: Interaction of small molecules with soluble and vesicle-bound αSyn. ( a ) Quantification of NMR signal intensities along the αSyn sequence when bound to SUVs in the absence (red line) and presence of a 15-fold excess of selegiline, EGCG, curcumin and baicalein (black bars). Signal intensities ( I ) were normalized by the values observed for αSyn in the absence of SUVs ( I 0 ). The lipid-to-protein molar ratio was 125:1. The ratio of NMR signal intensities of free (in the absence of SUVs) αSyn in the presence and absence of the respective compound are shown in light blue. ( b ) Chemical shift differences for free αSyn in the absence and presence of the compounds. EGCG causes intensity and chemical shift changes because of its binding to monomeric αSyn and conversion of αSyn into off-pathway oligomers. The dashed lines represent the intrinsic error for the chemical shift measurement. Full size image Interaction with Y39 and F94 drives NAC-domain release It was previously shown that PcTS directly binds to monomeric, soluble αSyn [34] . The interaction is driven by aromatic stacking with F4, Y39 and F94. In order to study the importance of Y39 and F94 for binding of PcTS to membrane-bound αSyn, we generated the αSyn mutants Y39A and F94A, as well as the double mutant Y39A/F94A. The SUV-induced intensity profiles of the mutants were similar to that of wild-type ( wt ) αSyn ( Fig. 6a–c ), indicating a similar affinity and mechanism of membrane binding. This was confirmed by determination of a dissociation constant of ~60±15 μM in all cases (assuming a one-site binding model; Fig. 5a ). It also suggests that Y39 and F94 are not important for anchoring αSyn to POPA/POPC vesicles, consistent with the observation that Y39 is primarily water-exposed when αSyn is bound to vesicles [44] . 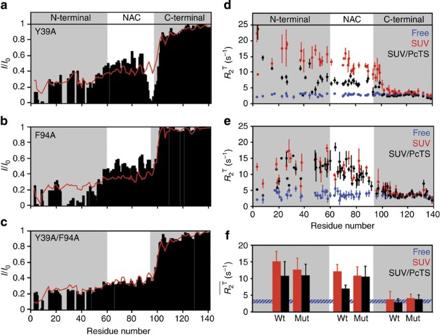Figure 6: Y39 and F94 are essential for PcTS-induced membrane detachment of αSyn. (a–c) Residue-specific NMR signal intensities in the αSyn variants (a) Y39A, (b) F94A and (c) Y39A/F94A in the presence of SUVs without (red line) and with a 15-fold excess (black bars) of PcTS. Signal intensities (I) were normalized by the values observed for each αSyn variant in the absence of SUVs (I0). The lipid-to-protein molar ratio was 125:1. White colour marks the aggregation-prone NAC region. In the absence of the two aromatic residues Y39 and F94, PcTS does not affect the binding of aSyn to vesicles. (d)15N R2Ttransverse spin-relaxation rates inwtαSyn in the absence of vesicles (blue), the presence of SUVs (red) and after further addition of a 15-fold excess of PcTS (black). The lipid-to-protein molar ratio was 6:1. In the presence of SUVs, the relaxation rates increase at the N terminus and the NAC region because of the exchange with the vesicle-bound state (red). PcTS-induced release of the NAC region increases the exchange between free and vesicle-bound αSyn causing a decrease inR2Tvalues (black). (e)15NR2Trates in the Y39A/F94A αSyn variant. Owing to the depletion of the binding sites, PcTS does not influence the exchange of this αSyn variant with membranes. As ind, error bars represent curve fitting errors. (f)R2Tvalues averaged over residues 1–60 (grey), 61–95 (white) and 96–140 (grey) in bothwtand Y39A/F94A (mut) αSyn. Values in the absence and presence of PcTS are shown by red and black bars. The average value ofR2Tin freewtαSyn is shown as blue horizontal line. Error bars indicate s.d. Figure 6: Y39 and F94 are essential for PcTS-induced membrane detachment of αSyn. ( a – c ) Residue-specific NMR signal intensities in the αSyn variants ( a ) Y39A, ( b ) F94A and ( c ) Y39A/F94A in the presence of SUVs without (red line) and with a 15-fold excess (black bars) of PcTS. Signal intensities ( I ) were normalized by the values observed for each αSyn variant in the absence of SUVs ( I 0 ). The lipid-to-protein molar ratio was 125:1. White colour marks the aggregation-prone NAC region. In the absence of the two aromatic residues Y39 and F94, PcTS does not affect the binding of aSyn to vesicles. ( d ) 15 N R 2 T transverse spin-relaxation rates in wt αSyn in the absence of vesicles (blue), the presence of SUVs (red) and after further addition of a 15-fold excess of PcTS (black). The lipid-to-protein molar ratio was 6:1. In the presence of SUVs, the relaxation rates increase at the N terminus and the NAC region because of the exchange with the vesicle-bound state (red). PcTS-induced release of the NAC region increases the exchange between free and vesicle-bound αSyn causing a decrease in R 2 T values (black). ( e ) 15 N R 2 T rates in the Y39A/F94A αSyn variant. Owing to the depletion of the binding sites, PcTS does not influence the exchange of this αSyn variant with membranes. As in d , error bars represent curve fitting errors. ( f ) R 2 T values averaged over residues 1–60 (grey), 61–95 (white) and 96–140 (grey) in both wt and Y39A/F94A ( mut ) αSyn. Values in the absence and presence of PcTS are shown by red and black bars. The average value of R 2 T in free wt αSyn is shown as blue horizontal line. Error bars indicate s.d. Full size image We then added PcTS to the αSyn variants in complex with vesicles. In the presence of a 15-fold excess of PcTS, NMR signal intensities in the NAC region of the Y39A mutant increased by ~15% ( Fig. 6a ), while the wt protein regained ~20–30% ( Fig. 3b,c ). In case of the F94A variant of αSyn, the PcTS-induced signal increase remained also below that of wt αSyn and was only slightly larger than for the Y39A mutant ( Fig. 6b ). Notably, simultaneous mutation of Y39 and F94 abolished the PcTS-induced signal increase in the NAC region ( Fig. 6c ). Thus, the partial release of αSyn’s NAC residues from the membrane surface is specifically because of the interaction of PcTS with Y39 and F94. To obtain further insight into the αSyn–membrane interaction, we performed 15 N spin relaxation measurements. Previous experiments had shown that the exchange with the membrane-bound α-helical state enhances the relaxation of the NMR resonances of disordered soluble αSyn [24] , [45] . Consistent with this finding, addition of SUVs increased the transverse 15 N spin relaxation rate from ~3 to 14 s −1 for residues 1–40 and to ~12 s −1 for residues 40–100 ( Fig. 6d ). In the presence of PcTS, relaxation rates in the N-terminal part of wt αSyn remained high, while in the NAC region the average 15 N transverse relaxation rate decreased from ~12 to 7 s −1 ( Fig. 6d,e ). The decreased contribution of the vesicle-bound state to the observed spin relaxation rate supports a PcTS-induced partial release of the NAC region of wt αSyn from the vesicle surface. In contrast, no PcTS-induced changes in relaxation rates were observed for the Y39A/F94A variant of αSyn ( Fig. 6e,f ), in agreement with the importance of Y39 and F94 for PcTS binding and NAC domain release. A distinct aggregation pathway of vesicle-bound αSyn Next, we asked whether the PcTS-mediated inhibition of aggregation of vesicle-bound αSyn ( Fig. 1 ) is connected to the PcTS-induced partial release of αSyn’s NAC region from the membrane surface ( Figs 3 and 6 ). To address this question, we analysed the influence of PcTS on the aggregation of both wt and mutant αSyn in the presence of vesicles ( Fig. 7 ). While PcTS completely blocked aggregation of vesicle-bound wt αSyn, the αSyn variants were able to form amyloid fibrils in the presence of PcTS ( Figs 1 and 7 ). Aggregation of the Y39A/F94A double mutant in the presence of PcTS even approached the aggregation behavior of wt αSyn in the absence of PcTS ( Fig. 7 ), despite the fact that its vesicle-induced broadening profile did not differ from that of wt αSyn ( Fig. 6c ). The slower fibrillization rate of the single point mutants when compared with Y39A/F94A αSyn ( Fig. 7a ) is in agreement with a PcTS-induced partial release of the NAC region of Y39A αSyn and F94A αSyn from the vesicle surface ( Fig. 6a,b ). The data demonstrate that membrane attachment of the NAC region is essential for aggregation of αSyn in a lipid environment. 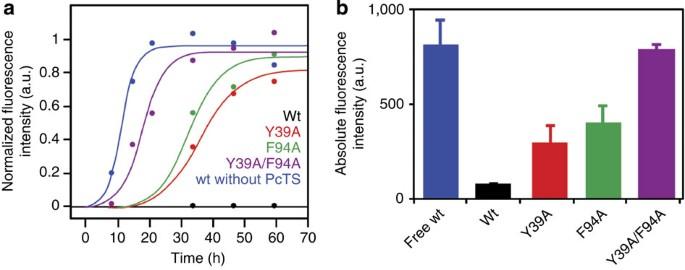Figure 7: Sequence specificity of small molecule-mediated inhibition of vesicle-bound αSyn amyloid formation. (a) Fibrillization kinetics ofwtαSyn and its mutants in the presence of a ~12.5mM concentration of SUVs. Shown is the normalized ThT intensity for increasing times of incubation in aggregation-prone conditions. The concentration of αSyn was 100 μM and the molar ratio of PcTS to protein was 15:1. The blue line shows the fibrillization kinetics ofwtαSyn in the absence of PcTS. In the presence of PcTS,wtαSyn (black) does not form ThT-positive fibrils. Removing one aromatic residue decreases the PcTS-inhibitory effect (green and red lines). Removal of both Y39 and F94 (purple line) largely abolishes the PcTS-mediated aggregation inhibition. The circles represent the average ThT intensity of at least three different experiments normalized against their respective maximum values. (b) ThT fluorescence after 6 days of aggregation. The error bars represent the s.e. of at least three different samples. Figure 7: Sequence specificity of small molecule-mediated inhibition of vesicle-bound αSyn amyloid formation. ( a ) Fibrillization kinetics of wt αSyn and its mutants in the presence of a ~12.5mM concentration of SUVs. Shown is the normalized ThT intensity for increasing times of incubation in aggregation-prone conditions. The concentration of αSyn was 100 μM and the molar ratio of PcTS to protein was 15:1. The blue line shows the fibrillization kinetics of wt αSyn in the absence of PcTS. In the presence of PcTS, wt αSyn (black) does not form ThT-positive fibrils. Removing one aromatic residue decreases the PcTS-inhibitory effect (green and red lines). Removal of both Y39 and F94 (purple line) largely abolishes the PcTS-mediated aggregation inhibition. The circles represent the average ThT intensity of at least three different experiments normalized against their respective maximum values. ( b ) ThT fluorescence after 6 days of aggregation. The error bars represent the s.e. of at least three different samples. Full size image It was previously shown that Y39 is important for αSyn aggregation in solution. When Y39 was mutated to alanine, the formation of fibrils was strongly delayed ( Fig. 8 ) [34] . Given the differences at the microenvironmental level between free and vesicle-bound αSyn, we asked whether the presence of this aromatic residue at position 39 plays a similar role for vesicle-bound αSyn. However, the Y39A mutation did not interfere with the aggregation of vesicle-bound αSyn ( Fig. 8 ). The distinct aggregation behaviour of the Y39A variant of αSyn in solution and when bound to vesicles demonstrates that the early stages of aggregation differ drastically between the free, disordered and the membrane-bound α-helical αSyn. 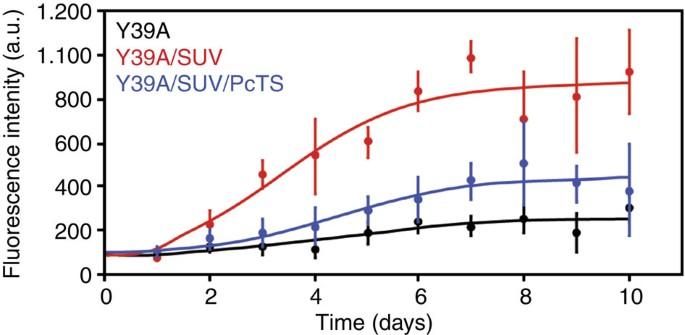Figure 8: Fibrillization kinetics of αSyn Y39A. Fibrillization kinetics of the Y39A mutant of αSyn in solution (black), when bound to membranes (red) and after further addition of PcTS (blue). Shown is the ThT fluorescence intensity after increasing times of incubation in aggregation-prone conditions (37 °C with stirring). The concentration of Y39A αSyn was 100 μM, that of SUVs ~12.5 mM. While little fibrillization was observed for the Y39A mutant of αSyn in solution, it readily aggregates in the presence of SUVs. Moreover, the data show that PcTS is capable of decreasing aggregation of vesicle-bound αSyn through an interaction with F94. Error bars represent the s.e. for at least three different samples. Figure 8: Fibrillization kinetics of αSyn Y39A. Fibrillization kinetics of the Y39A mutant of αSyn in solution (black), when bound to membranes (red) and after further addition of PcTS (blue). Shown is the ThT fluorescence intensity after increasing times of incubation in aggregation-prone conditions (37 °C with stirring). The concentration of Y39A αSyn was 100 μM, that of SUVs ~12.5 mM. While little fibrillization was observed for the Y39A mutant of αSyn in solution, it readily aggregates in the presence of SUVs. Moreover, the data show that PcTS is capable of decreasing aggregation of vesicle-bound αSyn through an interaction with F94. Error bars represent the s.e. for at least three different samples. Full size image PcTS reduces αSyn inclusion formation and cytotoxicity In order to determine the effect of PcTS on αSyn aggregation and αSyn-induced cytotoxicity, we employed a previously described cell model [46] that leads to protein inclusion formation positive for αSyn. Addition of 0.1 and 1 μM of PcTS to H4 cells expressing αSyn did not modify inclusion formation. In contrast, treatment with 10 μM PcTS for 48 h decreased the percentage of cells with inclusion formation ( Fig. 9a,b ). 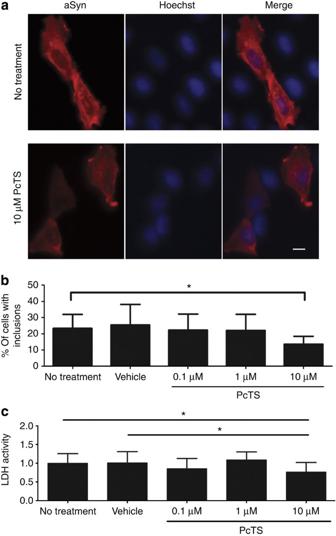Figure 9: PcTS reduces αSyn inclusion formation and cytotoxicity. (a) Representative images for αSyn inclusion modulation by 10 μM PcTS in H4 cells. Scale bar=25 μm. (b) Addition of 10 μM to H4 cells expressing αSyn decreases inclusion formation. No effect can be observed with lower concentrations of PcTS or vehicle control. (c) PcTS reduces αSyn-induced cytotoxicity. Addition of 10 μM PcTS to H4 cells expressing αSyn decreases release of LDH into the medium, an indicator for cytotoxicity. No effect could be observed with lower concentrations of PcTS or vehicle control. Data represent mean±s.d. of four or seven independent experiments withP<0.05 with paired, two-tailed Student’st-test and one-way analysis of variance withpost hocBonferroni. Figure 9: PcTS reduces αSyn inclusion formation and cytotoxicity. ( a ) Representative images for αSyn inclusion modulation by 10 μM PcTS in H4 cells. Scale bar=25 μm. ( b ) Addition of 10 μM to H4 cells expressing αSyn decreases inclusion formation. No effect can be observed with lower concentrations of PcTS or vehicle control. ( c ) PcTS reduces αSyn-induced cytotoxicity. Addition of 10 μM PcTS to H4 cells expressing αSyn decreases release of LDH into the medium, an indicator for cytotoxicity. No effect could be observed with lower concentrations of PcTS or vehicle control. Data represent mean±s.d. of four or seven independent experiments with P <0.05 with paired, two-tailed Student’s t -test and one-way analysis of variance with post hoc Bonferroni. Full size image Next, we tested whether PcTS would also influence αSyn-induced cytotoxicity in the same cell model. Toxicity was determined 48 h after transfection and start of PcTS treatment by determining the release of lactate dehydrogenase into the medium. We determined no effect on αSyn toxicity in the vehicle control, but observed a drop in LDH release upon treatment with 10 μM PcTS, the same concentration that led to inclusion modulation ( Fig. 9c ). αSyn is important for regulation of synaptic vesicle trafficking [8] and is found in both soluble and membrane fractions of neuronal cells [9] , [16] . Consistent with a physiological role of the membrane-bound conformation of αSyn, its N-terminal 100 residues have a high propensity to bind to negatively charged vesicles and fold into an α-helical conformation [25] , [47] . At the same time, αSyn can misfold, aggregate and form fibrils when it is in contact with phospholipid vesicles [38] pointing also to a pathological role of membrane-bound αSyn. Aggregation of vesicle-bound αSyn, which has a low surface coverage when compared with other peripheral membrane proteins such as apocytochrome c [44] , was suggested to occur through a two-state process [48] . Initially, the N terminus and the NAC domain of αSyn are bound to vesicles in an α-helical conformation. Aggregation is initiated by insertion of hydrophobic residues of the NAC domain into the membrane leading to an intermediate conformation. This intermediate conformation is at least partially inserted into the lipid bilayer and is characterized by partial unfolding of the helical conformation and formation of elements of β-structure [48] . A further step during aggregation of vesicle-bound αSyn is oligomerization through the NAC domain, which occurs either parallel to the unfolding of the helical conformation or subsequent to it [48] , followed by formation of amyloid fibrils. Amyloid fibrils formed in the presence of POPC/POPA vesicles closely resembled those formed in the absence of lipid vesicles and were immersed in a network of vesicles with substantially perturbed morphology [48] . A direct attachment of fibrils to SUVs is also supported by studies on the islet amyloid polypeptide, which showed that its fibrils line the surface of distorted phospholipid vesicles, in agreement with the notion that fibril growth at the membrane and membrane damage are physically connected [49] . Our data support the above aggregation model and reveal a way to interfere with aggregation of αSyn in contact with synaptic vesicles. PcTS directly binds to Y39 and F94 of membrane-bound αSyn. This interaction partially releases the NAC domain from the membrane surface ( Figs 3 and 6 ) such that the helical conformation in the NAC region is less prone to membrane-assisted unfolding, subsequent oligomerization and amyloid formation ( Figs 1 , 7 and 10 ). 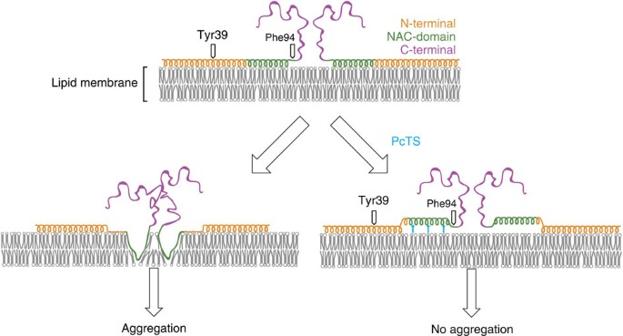Figure 10: Small molecule-mediated stabilization of helical vesicle-bound αSyn inhibits pathogenic aggregation. PcTS directly binds to vesicle-bound αSyn, stabilizes its helical conformation and delays misfolding and pathogenic aggregation. In contrast, EGCG, baicalein, curcumin and selegiline inhibit the conversion of the disordered monomeric αSyn into amyloid fibrils, but are not able to stabilize helical, vesicle-bound αSyn. Residues 1–60, 61–95 and 96–140 of αSyn are shown in orange, green and purple. Please see text for further details. Figure 10: Small molecule-mediated stabilization of helical vesicle-bound αSyn inhibits pathogenic aggregation. PcTS directly binds to vesicle-bound αSyn, stabilizes its helical conformation and delays misfolding and pathogenic aggregation. In contrast, EGCG, baicalein, curcumin and selegiline inhibit the conversion of the disordered monomeric αSyn into amyloid fibrils, but are not able to stabilize helical, vesicle-bound αSyn. Residues 1–60, 61–95 and 96–140 of αSyn are shown in orange, green and purple. Please see text for further details. Full size image Inhibition of αSyn aggregation in the membrane-bound state is specific to PcTS, since several other small molecules, which inhibit aggregation of αSyn in solution, did not stop aggregation in the lipid environment ( Fig. 10 ). This suggests that compounds such as curcumin and baicalein primarily act at the stage of soluble oligomer formation, while their affinity to monomeric αSyn is low. In addition, baicalein, selegiline and EGCG interact with liposomes ( Supplementary Fig. 2 ), further decreasing their efficacy in a lipid environment. PcTS, on the other hand, does not bind to liposomes and readily interacts with monomeric αSyn both in the absence and presence of lipid membranes. The green tea polyphenol EGCG also attenuated the formation of β-sheet-rich amyloid fibrils in the presence of vesicles, in agreement with its ability to bind to monomeric polypeptides [32] . However, in contrast to PcTS, EGCG was not able to stabilize the helical, membrane-bound conformation of αSyn ( Fig. 1 ). Instead, it directs αSyn into heterogeneous off-pathway oligomers [32] . It has also been demonstrated that, while EGCG is able to prevent the formation of aggregates and to disrupt already formed fibrils of the islet amyloid polypeptide when used in solution, its ability to do so in a phospholipid interface is greatly diminished [50] . Whether this is the result of a less accessible protein interface for the compound, membrane binding of EGCG or stabilization of the fibril by its interaction with phospholipids is unknown. The effectiveness of small molecules to inhibit aggregation of vesicle-bound proteins might also be related to changes in the aggregation pathway of the protein in the presence of lipids. Whatever the case, the combined data suggest that compounds, which show strong antiaggregation properties in solution, do not necessarily have the same efficacy when used in the presence of lipids. Thus, it is important to assess the antiaggregation properties of small molecules in a lipid environment, in particular as disruption of the cellular membrane might be a key mechanism how fibrillar/oligomeric species of αSyn acquire their neurotoxic properties. The fact that Y39 is essential for aggregation of αSyn in solution [34] but not when bound to membranes ( Fig. 8 ) shows that the very first stages of aggregation in a membrane environment are different from those that happen in solution. In solution the lack of an aromatic side chain in position 39 would interfere with the self-assembly process of aggregation, whereas in a membrane environment aggregation initially depends on the insertion of hydrophobic residues within the NAC domain and does not need aromatic residues for pathogenic aggregation [47] . PcTS inhibits the aggregation of prion proteins and has been investigated for its in vivo prophylactic and therapeutic effects in scrapie disease [42] . Inhibition of protease-resistant prion aggregates is achieved through stabilization of the native globular structure of the prion protein [51] . Thus, PcTS is able to stabilize well-folded protein conformations both in solution (prion protein) and on the membrane surface (αSyn; Fig. 1 ). PcTS is also likely to interfere with aggregation of membrane-bound β-synuclein, which has recently been shown to aggregate and cause neuronal loss in the rat brain [52] . β-synuclein binds membranes similar to αSyn and both Y39 and F94 are conserved [53] . Given the wide variety of models that have been proposed to explain the misfolding and aggregation of αSyn, the role of membrane interaction has generated mixed viewpoints. These range from the complete stabilization of the ‘native state’ of αSyn and inhibition of aggregation upon binding of αSyn to vesicles [9] , [16] , [17] , [54] to the formation of damaging pore-like oligomers formed only in the presence of membranes [39] . As part of these complex processes, αSyn maintains an equilibrium between a free and membrane-bound state and—under stress conditions—is prone to form soluble oligomers and fibrils. However, our study suggests that the mechanism by which αSyn aggregates is very different when it is bound to vesicles than when it is free in solution. We also demonstrate that the detachment of the NAC domain of αSyn from the vesicle surface greatly delays its aggregation and, to the best of our knowledge, this is a unique effect of PcTS. The importance of membrane attachment of the NAC domain for αSyn aggregation is consistent with a recent study, which showed that the NAC domain acts as a sensor of lipid properties and determines the affinity of αSyn membrane binding [25] . Because the antiaggregation effect of PcTS is much stronger for vesicle-bound αSyn than soluble, disordered αSyn, it is likely that PcTS reduces αSyn inclusion formation and cytotoxicity through binding to membrane-attached αSyn. Our study therefore suggests that small molecule-mediated stabilization of the helical membrane-bound state of αSyn provides unique opportunities for inhibiting misfolding and pathogenic aggregation of αSyn in the physiological environment of a synaptic vesicle. Detailed knowledge about the structural basis of αSyn aggregation, together with a screening procedure for small molecules that is targeted to helical vesicle-bound αSyn, promises new ways to approach Parkinson’s disease and related synucleinopathies. Expression and purification of αSyn variants pT7-7 plasmid encoding for human wt αSyn was kindly provided by the Lansbury Laboratory, Harvard Medical School, Cambridge, MA. A codon replacement was performed for residue Y136 (TAC to TAT) to avoid codon usage problems [55] . The resulting construct was then used as the template for mutagenesis reactions. Mutations were performed by using the QuikChange II site-directed mutagenesis kit (Stratagene) and verified by DNA sequencing. Plasmids containing αSyn variants were expressed in Escherichia coli BL21 (DE3) cells. Protein expression and purification was performed as previously described [56] . For production of 15 N-labelled proteins, M9-minimal medium supplemented with 15 NH 4 Cl (Cambridge Isotope Laboratories) was used. Preparation of unilamellar vesicles POPC and POPA, 1,2-dioleoyl- sn -glycero-3-phosphoethanolamine (DOPE), 1,2-dioleoyl- sn- glycero-3-phospho-L-serine (DOPS) and 1,2-dioleoyl- sn -glycero-3-phosphocholine (DOPC) were obtained from Avanti Polar Lipids. For vesicle formation, a 1:1 ratio of POPC:POPA or a 5:3:2 ratio of DOPE:DOPS:DOPC was dissolved in a 4-ml mixture of chloroform/methanol (1:1 vol/vol), followed by evaporation of all solvents under a stream of N 2 gas and lyophilized overnight. The resulting lipid film was hydrated in 50 mM HEPES, 100 mM NaCl, pH 7.4 or in 50 mM Na-phosphate buffer (pH 7.4), 100 mM NaCl to obtain a total lipid concentration of 12.5 mM. For preparation of SUVs, the suspension was sonicated at 37 kHz (four times for 10 min with 5 min breaks at room temperature or until the sample was transparent) in a glass tube. SUVs were isolated using ultracentrifugation at 55,000 r.p.m. in a Beckman TLA 100.3 rotor for 2 h at 298 K. The isolated SUVs had a hydrodynamic diameter of 35±10 nm according to dynamic light scattering. LUVs were prepared following the same procedure but with only two rounds of sonication and no ultracentrifugation step. Dynamic light scattering estimated the hydrodynamic diameter of the LUVs as 105±25 nm. Aggregation of vesicle-bound αSyn PcTS was purchased from MP Biomedicals (MP Biomedicals S.A., Heidelberg, Germany). Selegiline, curcumin, baicalein and EGCG were purchased from Sigma (Sigma-Aldrich Chemie GmbH, Schnelldorf, Germany). SUVs and LUVs were mixed with purified αSyn variants at a 125:1 molar ratio of phospholipid to protein in 50 mM HEPES, 100 mM NaCl pH 7.4, 0.02% sodium azide (with final concentrations of 12.5 mM of phospholipids and 100 μM for αSyn). All compounds were solubilized in a 500 mM stock solution of dimethyl sulfoxide and added to the working solution for final concentrations of 0.1, 0.5 and 1.5 mM (giving 1:1, 5:1 and 15:1 compound to protein ratios). Subsequently, samples were subjected to aggregation-prone conditions (37 °C ~300 r.p.m.) in low binding protein 1.5 ml Eppendorf tubes over a period of 10 days. After different incubation times, a 20-μl aliquot of the sample was mixed with 1 ml of a 100 mM ThT solution. Fluorescence emission was measured between 460 and 600 nm on a Varian Cary Eclipse fluorescence spectrophotometer (Agilent Technologies) with excitation wavelength of 442 nm at 20 °C. The averaged data points were fitted to a sigmoidal equation (data are presented as mean±s.e., n =3). CD spectroscopy Far UV-CD measurements were performed at 20 °C on a Chirascan (Applied Photophysics, UK) circular dichroism spectrometer, using a protein concentration of 10 μM in a quartz cuvette with 0.1-cm light path. For vesicle-bound αSyn, SUVs or LUVs were added to a final concentration of 1.5 mM. Each experiment was repeated at least twice. Baseline correction was performed with the same buffer. Data were expressed as the mean residue ellipticity (degree cm 2 d mol –1 ). Estimation of secondary structure content was performed by neural-network analysis using the programme K2D available at the DichroWeb server [57] . NMR spectroscopy NMR samples contained 0.1 mM 15 N-labelled wt or mutant αSyn in 50 mM HEPES buffer, 100 mM NaCl, pH 7.4 or 50 mM Na-phosphate buffer, 100 mM NaCl at pH 7.4 and 90% H 2 O/10% D 2 O. NMR experiments were recorded on a Bruker Avance 600 MHz spectrometer. The temperature was set to 15 °C. Data processing was performed using the software packages Topspin (Bruker) and CCPN Analysis [58] . To probe the binding of αSyn variants to vesicles, 2D 15 N– 1 H HSQC spectra were recorded in the presence of either 12.5 mM SUV or LUVs. The same stock solution of compounds in DMSO was used for the NMR experiments in the same ratios; therefore, the final DMSO concentration never surpassed 1% of the total volume. 15 N– 1 H HSQC amide cross-peaks affected during compound addition were identified by comparison of their chemical shift values with those of the same cross-peaks in the data set of samples lacking the compound. Perturbations in the chemical shift values for 1 H and 15 N were calculated as [(Δ δ 1 H) 2 +(Δ δ 15 N/10) 2 ] 1/2 . Intensity profiles ( I / I 0 ) were obtained by comparing intensities of 15 N– 1 H HSQC cross-peaks observed in the presence ( I ) and absence ( I 0 ) of compound. 15 N transverse relaxation optimized spectroscopy (TROSY) experiments for R 2 T measurement (modified from ref. 59 ) were recorded at 30 °C on a Bruker 600 MHz spectrometer as interleaved experiments with six T 2 delays (10, 40, 80, 150, 250 and 400 ms). Samples contained 250 μM protein and 1.5 mM SUVs (1:6 protein-to-lipid ratio) in 50 mM HEPES buffer, 100 mM NaCl at pH 7.4 with 10% D 2 O. Single exponential decay curves were fitted to the signal intensity of each cross-peak throughout the different delay times with the function y = Ae (− Bx ) + C , where B is the R 2 T value. Error bars represent the fitting errors. Transmission electron microscopy A solution containing protein was applied to glow-discharged carbon-coated grids and stained with 1% uranyl acetate. Images were taken in a Philips CM120 electron microscope (Philips Inc.) at a defocus of 2.3 μm using a TemCam 224 A slow scan CCD camera (TVIPS, Gauting, Germany). Cell culture and transfection H4 neuroglioma cells were maintained at 5% CO 2 and 37 °C in Optimem medium (Gibco) supplemented with 10% fetal calf serum and 1% Penicillin Streptomycin. One day before transfection cells were seeded in 24-well plates. Cells were transiently transfected with αSyn using Metafectene (Biontex) according to the manufacturer’s instructions. PcTS compound in DMSO was added in concentrations of 100 nM, 1 μM and 10 μM to the cells. αSyn-expressing cells were treated with DMSO to exclude vehicle effects. Immunocytochemistry Cells were fixed with 4% paraformaldehyde in PBS 48 h after transfection and start of PcTS treatment. For permeabilization cells were subsequently treated with 0.1% Triton X-100 and blocked with 1.5% bovine serum albumin (BSA) in PBS. Cells were then incubated with anti-αSyn antibody (BD 610787, 1:2,000) either 4 h at room temperature or overnight at 4 °C and 3 h in Alexa Fluor donkey anti-mouse 555 (Invitrogen A31570, 1:2,000). Cells were further stained with Hoechst (Molecular Probes 33258) for 5–10 min. Images were captured using a Leica DMI 6000B. LDH activity LDH activity was measured via release of LDH into the culture medium with the Cytotoxicity Detection Kit (LDH; Roche). Basic LDH release was measured in non-transfected cells, total LDH release was measured by cell lysis in 2% Triton X-100. Absorbance was measured with the Infinite M200 PRO (Tecan) plate reader at 490 nm. Experimental values were calculated in percentages of total LDH release and normalized to tranfection with SynT without treatment. Statistical analysis was conducted using GraphPad Prism 4.03 and included paired, two-tailed Student’s t -test. How to cite this article : Fonseca-Ornelas, L. et al. Small molecule-mediated stabilization of vesicle-associated helical α-synuclein inhibits pathogenic misfolding and aggregation. Nat. Commun. 5:5857 doi: 10.1038/ncomms6857 (2014).